Metformin improves healthspan and lifespan in mice Metformin is a drug commonly prescribed to treat patients with type 2 diabetes. Here we show that long-term treatment with metformin (0.1% w/w in diet) starting at middle age extends healthspan and lifespan in male mice, while a higher dose (1% w/w) was toxic. Treatment with metformin mimics some of the benefits of calorie restriction, such as improved physical performance, increased insulin sensitivity, and reduced low-density lipoprotein and cholesterol levels without a decrease in caloric intake. At a molecular level, metformin increases AMP-activated protein kinase activity and increases antioxidant protection, resulting in reductions in both oxidative damage accumulation and chronic inflammation. Our results indicate that these actions may contribute to the beneficial effects of metformin on healthspan and lifespan. These findings are in agreement with current epidemiological data and raise the possibility of metformin-based interventions to promote healthy aging. Metformin is a biguanide used since the 1960s in the treatment of type 2 diabetes and metabolic syndrome. It enhances insulin sensitivity, induces glycolysis and suppresses gluconeogenesis in the liver [1] , [2] , [3] . Patients with metabolic syndrome exhibit many manifestations of accelerated aging, such as cardiovascular disease, cancer and inflammatory disorders, all of which reduce lifespan. The fact that metformin treatment has been associated with reduced risk of cancer [4] and cardiovascular disease raises the possibility of a beneficial role of metformin for other age-related diseases [5] . Recently, we and others have studied pharmacological interventions that can delay aging and the incidence of age-related diseases [6] , [7] . Many of these interventions are based on the study of calorie restriction (CR) mimetics [8] , [9] . CR mimetics involve interventions that reproduce physiological and anti-aging effects found in CR animals. Several reports suggest that the actions of metformin resemble the effects of CR to some extent; microarray analyses have shown that metformin induces a gene expression profile that aligns with that of CR, although conflicting results have been shown in lifespan extension [9] , [10] , [11] , [12] , [13] , [14] , [15] . The mechanism of action of metformin involves, at least in part, activation of adenosine monophosphate-activated protein kinase (AMPK), an enzyme involved in cellular and whole-organism energy balance, as well as glucose and fat metabolism [16] , [17] . Separate evidence suggests that metformin may also act via AMPK-independent mechanisms [3] , [18] , [19] . The activation of AMPK is a well-known process triggered by an increase of the AMP/ATP ratio [20] . Several studies provide evidence that metformin partially inhibits complex I of the electron transport chain (ETC) with subsequent alteration of the mitochondrial performance, but the molecular mechanisms underlying this process have not been characterized in detail [21] , [22] , [23] . Thus, metformin may compromise ATP production in mitochondria leading to an increase of the AMP/ATP ratio. As a consequence of energy depletion, glycolysis is induced to maintain cellular metabolism. Even though mitochondrial poisons increase oxidative cellular damage by mechanisms involving increased reactive oxygen species [24] , [25] , there is no evidence that metformin induces the generation of reactive oxygen species and/or accumulation of oxidative damage [26] , [27] . In fact, the transcription factor SKN-1/Nrf2 is activated upon metformin treatment, resulting in increased expression of antioxidant genes in cells and animal models [10] . Reduced accumulation of oxidative damage may contribute to the inhibitory effects of metformin treatment in carcinogenesis models [3] , [28] , [29] . The ability of metformin to extend lifespan in the nematode Caenorhabditis elegans and the conflicting results in drosophila and mammals led us to study chronic metformin supplementation in laboratory mice [9] , [10] , [12] . Cohorts of middle-aged male C57BL/6 and B6C3F1 mice were provided with either a standard diet (SD) or SD supplemented with 0.1% (w/w) or 1% (w/w) metformin for the remainder of their lives. Our data show a level of chronic metformin exposure that leads to healthier and longer lives in mice, justifying further studies to determine if there is an exposure level that leads to improvement in healthspan and lifespan in humans. Metformin increases healthspan and longevity of mice We determined the long-term effects of two doses of metformin in male C57BL/6 mice. The first dose consisted of 0.1% metformin (w/w) supplemented in diet, which yielded a concentration of 0.45±0.09 mM in serum and 0.49±0.06 nmoles mg −1 protein in the liver. The second dose (1% w/w) yielded a concentration of 5.03±0.87 mM in serum and 3.67±0.32 nmoles mg −1 protein in the liver ( n =6–8 per group; age=84 weeks; diet=30 weeks; values presented as mean±s.e.m.). The survival curves of control and metformin-treated male mice separated shortly after the onset of the treatment. Diet supplementation with 0.1% metformin led to a 5.83% extension of mean lifespan ( Fig. 1a ), χ 2 =5.46 and P =0.02 in Gehan–Breslow survival test. In agreement with these data, a different strain of male mice (B6C3F1) supplemented with the same dose of metformin (0.1% w/w) resulted in a 4.15% extension of mean lifespan ( Supplementary Fig. S1 ), χ 2 =3.43 and P =0.064 in Gehan–Breslow survival test, which although is not significant suggests that the effects of metformin in longevity are not strain-specific. On the other hand, a higher concentration of the drug (1% w/w) was toxic and significantly shortened mean lifespan of C57BL/6 mice by 14.4% ( Fig. 1b ), likely owing to renal failure ( Supplementary Fig. S1 and Supplementary Table S1 ), χ 2 =51,70 and P <0.001 in Gehan–Breslow survival test. High doses of metformin have been associated with the development of lactic acidosis and the drug is contraindicated in patients with kidney dysfunction [30] . Importantly, male mice treated with 0.1% metformin in both longevity studies did not show any major difference in pathologies at 115 weeks of age nor obvious causes of death in the necropsies compared with SD-fed animals ( Supplementary Tables S1–S3 ). 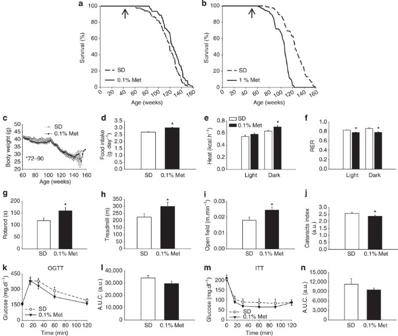Figure 1: Metformin increases survival and improves physical performance. (a,b) Kaplan–Meier survival curve for mice treated either with 0.1 or 1% metformin.n=64 for metformin 0.1% group andn=83 for their untreated counterparts;n=90 for metformin 1% group andn=88 for their untreated counterparts. The arrows at 54 weeks indicate the age at which metformin treatment was initiated. (c) Body weights. (d) Food consumption. (e,f)In vivometabolic response to 0.1% metformin treatment.n=9 per group. (e) Energy expenditure. (f) Respiratory exchange ratio. (g) Time to fall from an accelerating rotarod.n=16 per group. (h) Distance ran on treadmill performance.n=9 per group. (i) Average speed of animals in the open-field test.n=15–16 per group. (j) Metformin treatment delayed the onset of age-related cataracts.n=93–124 eyes per group. (k) Plasma levels of glucose after oral glucose load (OGTT).n=8 per group. (l) Area under OGTT curve. (m) Plasma levels of glucose after intraperitoneal insulin injection (ITT).n=9 per group. (n) Area under ITT curve. Met, metformin. Unless otherwise stated,n=all live animals in the study. Data are represented as the mean±s.e.m. *P<0.05 compared with SD-fed mice (t-test two tailed). Figure 1: Metformin increases survival and improves physical performance. ( a , b ) Kaplan–Meier survival curve for mice treated either with 0.1 or 1% metformin. n =64 for metformin 0.1% group and n =83 for their untreated counterparts; n =90 for metformin 1% group and n =88 for their untreated counterparts. The arrows at 54 weeks indicate the age at which metformin treatment was initiated. ( c ) Body weights. ( d ) Food consumption. ( e , f ) In vivo metabolic response to 0.1% metformin treatment. n =9 per group. ( e ) Energy expenditure. ( f ) Respiratory exchange ratio. ( g ) Time to fall from an accelerating rotarod. n =16 per group. ( h ) Distance ran on treadmill performance. n =9 per group. ( i ) Average speed of animals in the open-field test. n =15–16 per group. ( j ) Metformin treatment delayed the onset of age-related cataracts. n =93–124 eyes per group. ( k ) Plasma levels of glucose after oral glucose load (OGTT). n =8 per group. ( l ) Area under OGTT curve. ( m ) Plasma levels of glucose after intraperitoneal insulin injection (ITT). n =9 per group. ( n ) Area under ITT curve. Met, metformin. Unless otherwise stated, n =all live animals in the study. Data are represented as the mean±s.e.m. * P <0.05 compared with SD-fed mice ( t -test two tailed). Full size image Adult male C57BL/6 mice (from week 72 to 90) treated with 0.1% metformin were lighter than control animals ( Fig. 1c ). Mice on metformin tended to preserve body weight with advancing age, which has been associated with increased survival in rodent and human studies [31] , [32] . By 124 weeks of age, the average weight of metformin-treated mice was higher than SD-fed mice, although these observations were not found in B6C3F1 mice, probably because food intake in this strain was controlled ( Supplementary Fig. S1 ) [33] . Determinations of body composition during the lifetime of the animals revealed no significant differences in the percentage of fat mass and lean body mass or in the lean-to-fat ratio ( Supplementary Table S4 ). Although C57BL6/ mice fed with metformin were lighter, this group consumed more calories than their SD counterparts, indicating a shift in energy metabolism ( Fig. 1d ). The energy content of the faeces was identical in both groups, suggesting that metformin did not alter intestinal absorption of nutrients ( Supplementary Fig. S1 ). However, the beneficial effects of metformin might be explained, at least in part, by changes in the gut microbiota [34] , a process that has not been addressed in our study. Nevertheless, the effect of metformin on food consumption provides evidence against the possibility that metformin acts in a trivial fashion by leading to caloric restriction attributable to lack of palatability of metformin-supplemented chow. We next examined whether the increase in calorie intake was associated with higher energy expenditure. Indirect calorimetry revealed that metformin-treated animals showed higher heat production during the dark phase, when mice are normally more active ( Fig. 1e ). In accordance with previous reports demonstrating that metformin increases the use of lipids as a source of energy [35] , the respiratory exchange ratio was decreased during both the light and dark phases, and liver glyceride content was reduced in metformin-treated mice, indicating the preference for fat utilization ( Fig. 1f and Supplementary Fig. S1 ). Consistent with this hypothesis, β-oxidation of fatty acids was found to be increased while lipid synthesis was decreased in primary hepatocytes and mouse embryonic fibroblasts (MEFs) treated with metformin ( Supplementary Fig. S1 ). Interestingly, total levels of oxygen consumption and carbon dioxide production were not modified significantly by metformin in mice ( Supplementary Fig. S1 ). Moreover, there was no difference in spontaneous locomotion activity, suggesting that metformin shifts energy homeostasis of mice rather than their behaviour ( Supplementary Fig. S1 ). While the effect of metformin on longevity was obvious, it was important to determine whether the healthspan of the animals was preserved. We used several approaches to ascertain physical health of the animals. Rotarod, treadmill and open-field tests indicated that metformin improved the general fitness of laboratory mice ( Fig. 1g–i ). C57BL/6 mice are known to develop cataracts as they age [32] . Metformin supplementation led to significant reduction in lens opacity of 105-week-old mice ( Fig. 1j ), consistent with an overall improvement in healthspan. As mentioned earlier, metformin is widely prescribed to improve insulin sensitivity. Mice treated with 0.1% metformin showed lower glycated haemoglobin (Hb1Ac) levels 66 weeks after the treatment was initiated ( Table 1 ). Metformin-fed mice and mice on SD displayed comparable glucose homeostasis when measured by oral glucose tolerance test (OGTT) and insulin tolerance test (ITT) at 81 and 93 weeks of age, respectively ( Fig. 1k–n ). At 100 weeks of age, metformin-treated mice showed improvements in serum metabolite levels that are associated with diabetes compared with their control counterparts, with a reduction in insulin levels, total cholesterol, low-density lipoproteins and the homeostatic model assessment index-insulin resistance ( Table 1 ). Taken together, these results strongly suggest that metformin prevents the onset of metabolic syndrome. Table 1 Effects of 0.1% metformin treatment on various serum biomarkers. Full size table Metformin mimics CR transcriptome We have previously associated the induction of similar transcriptome to animals under CR in liver tissue, even in a 8-week treatment [15] . To test whether metformin shifts the physiology of ad lib -fed mice towards that of animals on CR after 30 weeks of treatment, we performed a genome-wide microarray analysis on liver and muscle tissues of three groups of mice ad lib -fed with SD, 0.1% metformin or CR. Principal component analysis (PCA) demonstrated a clear effect of metformin treatment, with the global gene expression profile shifting towards the changes induced by CR ( Fig. 2a ). According to a previous report, further analysis of the transcript profile revealed that the majority of the genes whose expression was modified by CR and 0.1% metformin were shifted in the same direction in the liver and muscle ( Fig. 2b ) [15] . Of these, expression of the cytokine-inducible SH2-containing protein ( CISH ) gene, which belongs to the cytokine-induced STAT inhibitor family [27] , was one of the most highly induced genes found in the liver and muscle of metformin- and CR-treated mice ( Supplementary Table S5 ). Under the metformin and CR regimen, the expression of serum amyloid protein genes ( Saa1 and Saa2 ) was markedly decreased in the liver, suggesting the suppression of inflammatory responses [36] . 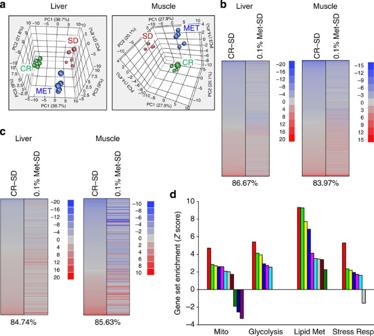Figure 2: Metformin shifts expression patterns of mice towards those on calorie restriction. (a) PCA was performed on differentially expressed genes from the liver and muscle tissue of mice maintained on SD and 0.1% metformin. Each data point corresponds to the PCA analysis of each subject. (b) Gene expression profile comparing genes significantly upregulated (red) and downregulated (blue) by either CR or metformin compared with SD mice (z-ratio). The percentage of significant gene expression changes shifted in the same direction in CR and metformin treatments compared with SD mice is presented in brackets. (c) Comparison of gene sets significantly altered by CR and metformin treatment compared with SD expression (z-score); upregulated (red) and downregulated (blue) gene sets. The percentage of significant gene sets changes shifted in the same direction in CR and metformin treatments compared with SD mice is presented in brackets. (d) Effect of metformin on mitochondria (Mito), glycolysis, lipid metabolism (Lipid Met) and stress response (Stress Resp)-related gene sets. The list of all the significantly modified gene sets can be found inSupplementary Table S6. Met, metformin. Figure 2: Metformin shifts expression patterns of mice towards those on calorie restriction. ( a ) PCA was performed on differentially expressed genes from the liver and muscle tissue of mice maintained on SD and 0.1% metformin. Each data point corresponds to the PCA analysis of each subject. ( b ) Gene expression profile comparing genes significantly upregulated (red) and downregulated (blue) by either CR or metformin compared with SD mice ( z -ratio). The percentage of significant gene expression changes shifted in the same direction in CR and metformin treatments compared with SD mice is presented in brackets. ( c ) Comparison of gene sets significantly altered by CR and metformin treatment compared with SD expression ( z -score); upregulated (red) and downregulated (blue) gene sets. The percentage of significant gene sets changes shifted in the same direction in CR and metformin treatments compared with SD mice is presented in brackets. ( d ) Effect of metformin on mitochondria (Mito), glycolysis, lipid metabolism (Lipid Met) and stress response (Stress Resp)-related gene sets. The list of all the significantly modified gene sets can be found in Supplementary Table S6 . Met, metformin. Full size image We used parametric analysis of gene-set enrichment (PAGE) analysis to further highlight functional pathways modified in response to 0.1% metformin and CR. Both interventions led to a significant overlap in the number of upregulated and downregulated gene sets present in the liver (84.7%) and muscle (85.6%), supporting that metformin closely mimics the CR transcriptome ( Fig. 2c ) [15] . The liver has a central role in the maintenance of glucose homeostasis and has been proposed as one of the main targets of metformin [37] . In the livers of metformin-treated mice, PAGE analysis showed a significant alteration in 220 gene sets ( Supplementary Table S6 ), many of these were related to mitochondrial function, glycolysis, lipid biosynthesis and stress response ( Fig. 2d ). In accordance with microarray data, quantitative PCR indicated the increase in the mRNA levels of several genes encoding transcriptional regulators and enzymes involved in mitochondrial energetics, glycolysis and fatty acid metabolism ( Supplementary Fig. S2 ). Moreover, there was a significant downregulation of gene sets related to autophagy, apoptosis and ubiquitin cycle in the liver of metformin-fed mice. Several stress response pathways were induced by metformin as shown by Ingenuity Pathway Analysis ( Supplementary Fig. S3 ). Nrf2 is a transcription factor that regulates the expression of multiple antioxidant genes and is also required for the beneficial effects of metformin in C. elegans [10] . Here, metformin treatment also induced Nrf2 target gene activation. The overall interpretation of these results is that metformin exerts CR-like genomic and metabolic responses by inducing longevity-associated pathways in laboratory mice. Preservation of mitochondrial function by metformin It has been proposed that mild inhibition of the mitochondrial ETC complex I activity by metformin [21] , [22] reduces ATP production and contributes to increase the AMP/ATP ratio, which, in turn, results in AMPK activation. AMPK has an important role in the regulation of energy metabolism [38] . In cultured MEFs and in livers of treated mice, metformin increased the relative levels of phosphoactive AMPK (Thr172) by 27% ( P <0.05, t -test two tailed), which led to increased phosphorylation at Ser-79 of its direct target, acetyl-CoA carboxylase, by 169% ( P <0.01, t -test two tailed) ( Fig. 3a,b , Supplementary Fig. S4 , Supplementary Tables S7 and S8 for entire western blot images and densitometric analyses). The ATP content in the liver of metformin-treated mice was unaffected, which may stem from increased hepatic glycolysis ( Supplementary Fig. S5 ). In parallel, we examined mitochondrial performance in cultured MEFs in response to metformin ( Fig. 3c ) and found a decrease in oxygen consumption rate, in agreement with earlier reports [39] . Oxygen consumption was also decreased following the addition of the mitochondrial uncoupler, carbonyl cyanide-4-(trifluoromethoxy)phenylhydrazone, which indicates that metformin altered maximal oxygen consumption in MEFs. Cell culture media showed a reduction in pH on exposure of cells to metformin ( Supplementary Fig. S5 ), which is consistent with reports showing increased lactic acid production due to an increase in glycolysis and studies that associate the risk of lactic acidosis to metformin administration to diabetic patients [40] . Furthermore, metformin induced the expression of cytosolic lactate dehydrogenase, the enzyme responsible for lactic acid production, both in MEFs and in the liver of treated animals ( Supplementary Fig. S5 ). 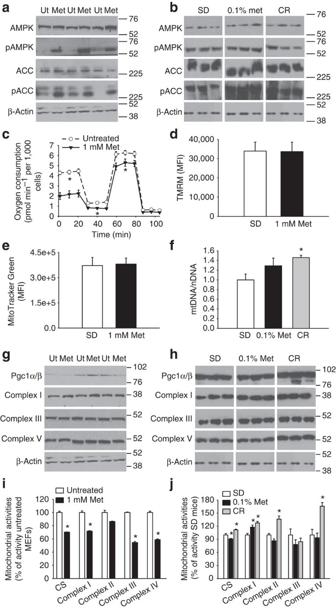Figure 3: Metformin activates AMPK without alteringin vivoETC activities. (a) Activation of AMPK by metformin in MEFs. AMPK and acetyl-coA carboxylase (ACC) phosphorylation by metformin.n=3 per group. (b) Activation of AMPK and ACC phosphorylation in the liver of 0.1% metformin-treated mice.n=4–6 per group. (c) Oxygen consumption in MEFs treated with 1 mM metformin.n=3 per group. (d,e) Mitochondrial content in MEFs treated with metformin was determined by TMRM (d) and MitoTracker green (e) staining, MFI, mean fluorescence intensity.n=3 per group. (f) Mitochondrial DNA content analysed by quantitative PCR in the liver.n=5–8 per group. (g) Mitochondrial protein levels in MEFs treated with metformin.n=3 per group. (h) Mitochondrial protein levels in the liver from 0.1% metformin-treated mice.n=4–6 per group. (i,j) Effect of metformin on mitochondrial enzymatic activities. (i) MEFs treated with 1 mM metformin (n=3 per group) and (j) liver lysates from 0.1% metformin-treated mice (n=5–6 per group). Met, metformin; Ut, untreated. Data are represented as the mean±s.e.m. *P<0.05 versus untreated controls or SD-fed mice (t-test two tailed). Figure 3: Metformin activates AMPK without altering in vivo ETC activities. ( a ) Activation of AMPK by metformin in MEFs. AMPK and acetyl-coA carboxylase (ACC) phosphorylation by metformin. n =3 per group. ( b ) Activation of AMPK and ACC phosphorylation in the liver of 0.1% metformin-treated mice. n =4–6 per group. ( c ) Oxygen consumption in MEFs treated with 1 mM metformin. n =3 per group. ( d , e ) Mitochondrial content in MEFs treated with metformin was determined by TMRM ( d ) and MitoTracker green ( e ) staining, MFI, mean fluorescence intensity. n =3 per group. ( f ) Mitochondrial DNA content analysed by quantitative PCR in the liver. n =5–8 per group. ( g ) Mitochondrial protein levels in MEFs treated with metformin. n =3 per group. ( h ) Mitochondrial protein levels in the liver from 0.1% metformin-treated mice. n =4–6 per group. ( i , j ) Effect of metformin on mitochondrial enzymatic activities. ( i ) MEFs treated with 1 mM metformin ( n =3 per group) and ( j ) liver lysates from 0.1% metformin-treated mice ( n =5–6 per group). Met, metformin; Ut, untreated. Data are represented as the mean±s.e.m. * P <0.05 versus untreated controls or SD-fed mice ( t -test two tailed). Full size image Our microarray and quantitative PCR analyses showed increased expression of several mitochondrial genes in the livers of metformin-treated mice. However, metformin lowered oxygen consumption in MEFs, suggesting that these alterations in mitochondrial bioenergetic function may occur in cell cultures. The administration of this anti-diabetic drug did not alter several markers of mitochondrial content in both MEFs and the liver of treated mice ( Fig. 3d–f ), while causing only moderate increase, if any, in the expression of several subunits in the ETC complexes ( Fig. 3g,h ). Among key enzymes of the tricarboxylic acid cycle and ETC that were assayed, complex I activity was significantly lower in metformin-treated MEFs ( Fig. 3i ). In contrast, mice treated with metformin had a remarkable increase in hepatic complex I activity ( Fig. 3j ). The activity for complexes III and IV was significantly reduced by metformin in MEFs, but remained unchanged in liver lysates of metformin-treated mice. The differential effects of metformin in vitro and in vivo may be owing to the hepatocytes adapting to long-term inhibition of complex I activity. Interestingly, and in agreement with our findings, preservation of mitochondrial complex I activity, at least in muscle, has been recently reported after long-term metformin treatment in humans [41] . Furthermore, the inhibition of mitochondrial respiration by metformin is reported to be concentration-dependent, with no effect at concentrations lower than 1 mM [42] . Serum level of metformin was 0.45±0.09 mM (mean±s.e.m.) in 0.1% metformin-treated mice, which is considerably higher than seen in the serum of diabetic patients treated with metformin [43] , but lower than those used in most in vitro models that demonstrate inhibition of mitochondrial respiration by this compound [21] , [22] , [42] . The degree of inhibition of oxidative phosphorylation as a function of metformin serum levels cannot be quantitated because of the fact that active uptake of metformin occurs via transporters on the cell surface and, possibly, mitochondria. Metformin inhibits chronic inflammation The activation of the SKN-1/Nrf2-dependent antioxidant response is required for the beneficial effects of metformin in C. elegans [10] . There was a trend towards reduction in superoxide production in mitochondrial complexes in the livers of metformin-treated mice ( P =0.09, t -test two tailed) ( Supplementary Fig. S6 ). When divided by the total activity of mitochondrial complexes I–II to III, the proportion of superoxide leakage was significantly decreased by metformin ( Fig. 4a ), indicating greater efficiency of mitochondrial complexes in transferring electrons to their expected acceptors in the ETC. Moreover, the marked reduction in the amount of lysine-4-hydroxynonenal-modified proteins and 8-iso-PGF2α, a marker of lipid peroxidation, was consistent with decreased oxidative stress damage in the liver of metformin-treated mice ( Fig. 4b,c ). To investigate whether metformin activates the Nrf2-dependent antioxidant response, HepG2 cells stably expressing a Nrf2-responsive antioxidant response element (ARE) luciferase reporter construct were treated with increasing concentrations of metformin for 16 h ( Fig. 4d ). The increase in Nrf2/ARE reporter activity occurred with an ED 50 of ~1.5 mM metformin without reduction in cell survival ( Supplementary Fig. S6 ). The cellular reduction of the tetrazolium dye MTT (3-(4,5-dimethylthiazol-2-yl)-2,5-diphenyltetrazolium bromide), an assay that measures NADH oxidase activity, was lower in metformin-treated cells, with an IC 50 of ~3.3 mM ( Supplementary Fig. S6 ). Finally, in the livers of treated mice, 0.1% metformin contributed to an increase in the level of antioxidant and stress response proteins, including SOD2, TrxR1, NQO1 and NQO2 ( Fig. 4e ), further contributing to the reduction in hepatic oxidative stress damage. 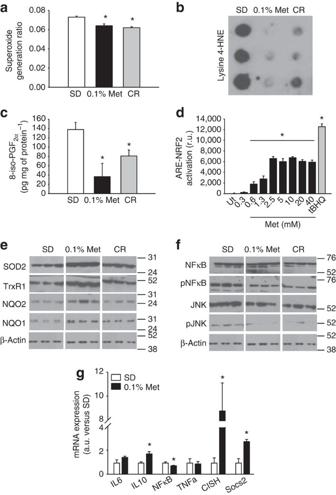Figure 4: Metformin enhances antioxidant defenses and inhibits inflammation. (a) Rate of electrons derived to superoxide generation in mitochondrial complexes I and II to III in the liver of 0.1% metformin-treated mice.n=5–6 per group. (b) Oxidative damage in proteins determined by lysine-4-hydroxinonenal levels in the liver of 0.1% metformin-treated mice (n=4–6 per group). (c) Oxidative damage in lipids determined by 8-iso-PGF2αlevels in the liver of 0.1% metformin-treated mice (n=4–6 per group). (d) Nrf2–ARE assay determining Nrf2–ARE-dependent expression in metformin-treated HepG2 cells. tBHQ was added as positive control for NRF2–ARE induction (n=3 per group). (e) Antioxidant and stress response protein levels in the liver of 0.1% metformin-treated mice (n=4–6 per group). (f) Activation of pro-inflammatory signalling pathways in the liver of 0.1% metformin-treated mice (n=4–6 per group). (g) Expression of multiple inflammatory-related genes in the liver of 0.1% metformin-treated mice (n=5 per group). Met, metformin. Data are represented as the mean±s.e.m. *P<0.05 versus SD-fed mice (t-test two tailed). Figure 4: Metformin enhances antioxidant defenses and inhibits inflammation. ( a ) Rate of electrons derived to superoxide generation in mitochondrial complexes I and II to III in the liver of 0.1% metformin-treated mice. n =5–6 per group. ( b ) Oxidative damage in proteins determined by lysine-4-hydroxinonenal levels in the liver of 0.1% metformin-treated mice ( n =4–6 per group). ( c ) Oxidative damage in lipids determined by 8-iso-PGF 2α levels in the liver of 0.1% metformin-treated mice ( n =4–6 per group). ( d ) Nrf2–ARE assay determining Nrf2–ARE-dependent expression in metformin-treated HepG2 cells. tBHQ was added as positive control for NRF2–ARE induction ( n =3 per group). ( e ) Antioxidant and stress response protein levels in the liver of 0.1% metformin-treated mice ( n =4–6 per group). ( f ) Activation of pro-inflammatory signalling pathways in the liver of 0.1% metformin-treated mice ( n =4–6 per group). ( g ) Expression of multiple inflammatory-related genes in the liver of 0.1% metformin-treated mice ( n =5 per group). Met, metformin. Data are represented as the mean±s.e.m. * P <0.05 versus SD-fed mice ( t -test two tailed). Full size image The development of chronic inflammation is one of the hallmarks of oxidative damage accumulation. Inflammatory processes contribute to liver dysfunction in aging and are known to be suppressed by CR [44] . In this context, increases in the relative levels of phosphoactive forms of NF-κB and JNK have been shown to contribute to pro-inflammatory signalling [45] , [46] . Interestingly, metformin reduces the production of inflammatory markers in human liver cells [36] . In the livers of metformin-treated mice, a decline in pNF-κB by 64% ( P <0.01, t -test two tailed) and pJNK by 79% ( P <0.01, t -test two tailed) levels was observed ( Fig. 4f ) together with attenuated expression of NF-κB gene ( Fig. 4f ). An additional gene expression signature associated with metformin treatment was the increased expression of several anti-inflammatory genes ( Fig. 4g ). These results are in agreement with the fact that metformin reduces the number of activated macrophages, although we could not detect significant differences in the number of infiltrated macrophages in the liver of the mice ( Supplementary Fig. S6 ). Further research will be required to address this fact. In summary, the ability of metformin to reduce oxidative stress and inflammation suggests that this could partly be the reason why this drug confers health and lifespan benefits in laboratory mice. Our model reveals a level of chronic metformin exposure that lengthens lifespan and also attenuates the deleterious effects of aging in male mice. The effects of metformin resembled to some extent the effects of caloric restriction, even though food intake was increased. While it is clear that in short-term in vitro models metformin partially inhibits oxidative phosphorylation, we find no evidence for this with long-term exposure in vivo , suggesting that adaptation to metformin occurs, and is associated with benefits, including reduced oxidative stress and increased antioxidant defenses, leading to lower oxidative damage accumulation and inhibition of chronic inflammation. The dose associated with these beneficial effects was well tolerated in mice, but lead to serum levels an order of magnitude higher than those conventionally used in treatment of diabetes in human patients. Thus, while the pleotropic effects of metformin in vivo presents challenges in the identification of the specific mechanisms that are critical for the observed improvements on health and aging, pharmacokinetic issues must be addressed before results from our model can be extrapolated to other species. Further studies are required to determine the effects of chronic exposure levels to biguanides in health and aging in humans. Animal models and diets Animal procedures, housing and diets were in accordance with the guidelines issued by the Intramural Research Program of the National Institutes of Health protocol number 352TGB2013. Male C57BL/6 mice at either 6 months of age (for 0.1% metformin and CR) or 11 months of age (for 1% metformin dose) were purchased from the National Institute on Aging Aged Rodent Colony from Charles River. The C57BL/6 mice were maintained on a standard purified mouse diet (AIN-93G) until they reached 1 year of age when the treatments started. The CR animals were subjected to a lifelong restriction on AIN-93G diet, starting at 27 weeks of age, with a daily food allotment of 60% of that eaten by the ad lib animals. Besides CR animals, the C57BL/6 groups in this study were fed the standard AIN-93G diet (SD) or AIN-93G plus 0.1% metformin or 1% metformin ad lib for the remainder of their lives. Pure metformin was obtained from Farmhispania (Farmhispania S.A., Barcelona, Spain) and mixed to homogeneity during manufacturing of the diets (Dyets Inc., Bethlehem, PA). For B6C3F1 mice longevity study, male mice (Harlan Breeders, Indianapolis) were randomly assigned to treatment groups at 12 months of age. In the control group, mice were shifted from ad lib chow feeding (Diet # 5001, Purina Mills, Richmond, IN) to daily feeding with 13.3 kcal per day per mouse of control diet (AIN-93M, Diet No. F05312; BioServ, Frenchtown, NJ). For the metformin B6C3F1 group, mice were shifted to daily feeding with an identical quantity of control AIN-93M diet supplemented with metformin (Caraco Pharmaceutical Laboratories, Detroit, MI) at 100 mg kg −1 diet (0.1% w/w) (~10.6 mg kg −1 bw per day. All mice were fed daily and, with rare exceptions, all food was eaten each day. Metformin was mixed with powdered diet and cold pressed into 1-g pellets by BioServ. The chow was produced every 3 months during the length of the study, never was permitted to exceed 50 °C and was kept away from light whenever possible to ensure the stability of metformin (the light/dark cycle in the mouse facility was not altered). Stock metformin and all chow were stored in the dark at 4 °C. The mice were on a light:dark 12:12-h schedule and maintained between 20–22 °C according to animal protocols and NIH guidelines. Food intake and body weight were measured on a biweekly or bimonthly basis for the duration of the study. Survival curves were plotted using the Kaplan–Meier method, which includes all available animals at each time point. The criteria for euthanasia was based on an independent assessment by a veterinarian, according to AAALAC guidelines and only cases, where the condition of the animal was considered incompatible with continued survival, are represented in the curves. Every animal found dead or euthanized was necropsied for pathology score. The C57BL/6 0.1% metformin group started with 64 mice and the corresponding 83 corresponding SD control mice. CR group: 76 mice. The C57BL/6J 1% metformin group: 90 mice; SD-matched group: 88 mice. The B6C3F1 0.1% metformin group: 36 mice; SD-matched group: 297 mice. Faecal analysis Total energy in faeces was determined in 0.6±0.04 g of faecal samples in a 1281 Oxygen Bomb Calorimeter (Parr Instrument, Moline, IL) according to the manufacturer’s protocol. ( n =3–5 per group; age=66 weeks; diet=12 weeks). Metabolic clamps Mouse metabolic rate was assessed by indirect calorimetry in open-circuit oxymax chambers using the Comprehensive Lab Animal Monitoring System (CLAMS; Columbus Instruments, Columbus, OH). Mice were housed singly with water and food available ad lib , except for CR group, and maintained at 20–22 °C under a 12:12-h light–dark cycle (light period 0600–1800 hours). All mice were acclimatized to monitoring cages for 3–6 h before recording. Sample air was passed through an oxygen sensor for determination of oxygen content. Oxygen consumption was determined by measuring oxygen concentration in air entering the chamber compared with air leaving the chamber. The sensor was calibrated against a standard gas mix containing defined quantities of oxygen, carbon dioxide and nitrogen. Constant airflow (0.6 l min −1 ) was drawn through the chamber and monitored by a mass-sensitive flowmeter. The concentrations of oxygen and carbon dioxide were monitored at the inlet and outlet of the sealed chambers to calculate oxygen consumption. Measurement in each chamber was recorded for 30 s at 30-min intervals for a total of 60 h. The second dark:light cycle is represented in the plots. Movement (both horizontal and vertical) was also monitored. The system has beams 0.5 inches apart on the horizontal plane, providing a high-resolution grid covering the XY planes and the software provides counts of beam breaks by the mouse in 30-s epochs ( n =9 per group; age=71 weeks; diet=17 weeks). Physical performance tests Results from rotarod, treadmill and open-field are presented as follows: time to fall from an accelerating rotarod (4–40 r.p.m. over 5 min); total distance ran in the treadmill test until exhaustion; and the speed of the animals in the open-field. Rotarod: mice were given a habituation trial on day 1 where they were placed on the rotarod at a constant speed (4 r.p.m.) and had to remain on the rotarod for 1 min. Results shown are the average of three trials per mouse, measuring time to fall from an accelerating rotarod (4–40 r.p.m. over 5 min). The maximum trial length was 5 min, and there was a 30-min rest period between each trial ( n =16 per group; age=95 weeks; diet=41 weeks). For the treadmill test, mice were required to exercise on the treadmill until exhaustion. The treadmill was horizontal (0° incline) and mice ran in groups of six. Subjects were habituated at a constant speed of 4 m min −1 for 5 min. The following day, each mouse was given a trial starting at 7 m min −1 for 0–3 min, 12 m min −1 for 3–7 min, 15 m min −1 for 7–25 min and 19 m min −1 for 25 min ( n =9 per group; age=73 weeks; diet=19 weeks). For open-field determinations, mice were placed on the field and movement was recorded for 300 s using Field 2020 tracking software from HVS Image. Results were averaged for movement speed ( n =15–16 per group; age=95 weeks; diet=41 weeks). Insulin, OGTT and ITT To determine glucose and insulin levels, blood samples were collected by venipuncture and analysed as described in Supplementary Information [7] . Serum markers and hormones Serum metabolites were quantified using a COBAS Integra 400 instrument according to the manufacturer’s instructions (Roche, Indianapolis, IN). HbA1c levels were determined according to the manufacturer’s protocol using the mouse HbA1c kit (Crystal Chem, Downers Grove, IL). Microarray analysis RNA from tissues was isolated using the RNeasy kit (Qiagen, Valencia, CA) and then hybridized to BD-202-0202 Illumina Beadchips. Raw data were subjected to Z -normalization, as described elsewhere [47] , [48] . PCA, performed on the normalized Z -scores of all of the detectable probes in the samples, was performed by using the DIANE 6.0 software ( http://www.grc.nia.nih.gov/branches/rrb/dna/diane_software.pdf ). Significant genes were selected by the z -test <0.05, false discovery rate <0.30, as well as z -ratio >1.5 in both directions and analysis of variance P- value <0.05. PAGE was analysed as previously described [49] . Gene regulatory network and canonic pathway analysis was performed by using Ingenuity Pathway Analysis. Oxygen consumption Oxygen consumption in MEFs was measured using the Seahorse 24 × F instrument (Seahorse Biosciences, North Billerica, MA). In brief, cells were seeded into Seahorse tissue culture plates and treated without or with 1 mM metformin for 16 h. Then, the medium was changed and the assay was run. A detailed explanation of the protocol is included in Supplemental Information. Nrf2/ARE pathway activity Nrf2 induction was determined according to the manufacturer’s protocols (Invitrogen, La Jolla, CA). A detailed explanation of the protocols is described in Supplementary Information . Mitochondrial mass determination MEFs (2 × 10 6 ) were seeded in a 100-mm culture dish. After 24 h, cells were washed once in PBS, trypsinized and then resuspended in phenol red-free DMEM supplemented with 10% fetal bovine serum containing either 50 nM MitoTracker Green FM (Invitrogen) or 20 nM tetramethyl rhodamine methyl ester (TMRM) (Invitrogen). Cells stained with TMRM were incubated for 15 min at 37 °C while 30-min incubations were used for MitoTracker Green FM. Fluorescence was measured by a flow cytometer (C6 Flow Cytometer, Accuri, MI). Superoxide generation Superoxide production was determined in liver samples by the reduction of acetylated cytochrome c [50] according to a method described previously for succinate:NADH-cytochrome c reductase with minor modifications [51] . Lipid peroxidation Lipid peroxidation was determined by quantifing the levels of 8-iso-prostaglandin F 2α according to the manufacturer’s protocol using the 8-iso-PGF 2α ELISA kit (Enzo Life Sciences, Farmington, NY). Body composition Several times during the length of the study, the amounts of body fluid, fat and lean body mass were determined in whole live mice. The assessment was acquired by NMR using the Minispec LF90 (Bruker Optics, Billerica, MA). Statistical analysis Unless otherwise stated, Student’s t -test two tailed assuming unequal variances was used. Analyses were performed using Excel 2010 (Microsoft Corp., Redmond, WA). For longevity studies, Gehan–Breslow statistical test was used and analyses were performed using sigmastat 3.5 (Systat Software Inc., San Jose, CA). Microarray data are accessible in GEO database under accession code GSE40936 . In all experiments, results are represented as the mean±s.e.m. In all cases, P -values ≤0.05 were considered significant. Accession codes: Microarray data have been deposited in the Gene Expression Omnibus database under accession code GSE40936 . How to cite this article: Martin-Montalvo A. et al . Metformin improves healthspan and lifespan in mice. Nat. Commun. 4:2192 doi: 10.1038/3192 (2013).